Experimental evidence of replica symmetry breaking in random lasers Spin-glass theory is one of the leading paradigms of complex physics and describes condensed matter, neural networks and biological systems, ultracold atoms, random photonics and many other research fields. According to this theory, identical systems under identical conditions may reach different states. This effect is known as replica symmetry breaking and is revealed by the shape of the probability distribution function of an order parameter named the Parisi overlap. However, a direct experimental evidence in any field of research is still missing. Here we investigate pulse-to-pulse fluctuations in random lasers, we introduce and measure the analogue of the Parisi overlap in independent experimental realizations of the same disordered sample, and we find that the distribution function yields evidence of a transition to a glassy light phase compatible with a replica symmetry breaking. Replica theory was originally introduced by Edwards and Anderson and detailed by Sherrington and Kirkpatrick to try to solve the prototype model for spin-glasses [1] . It was readily recognized as one of the fundamental paradigms of statistical mechanics and, after Parisi resolution of the mean-field theory [1] , found applications in a huge variety of different fields of research [2] , [3] . Spin-glass theory gives a rigorous settlement to the physical meaning of complexity, and describes a number of out-of-equilibrium phenomena (for example, weak non-ergodicity and aging) [1] , [4] . More recently this theory has found application in the field of random photonics [5] , as specifically for random lasers (RLs) and nonlinear waves in disordered systems [6] , [7] , [8] . However, notwithstanding the theoretical relevance, an experimental demonstration of the most important effect, the so-called replica symmetry breaking (RSB) is still missing. Spin-glass theory predicts that the statistical distribution of an order parameter, the Parisi overlap, changes shape when a large number of competing equilibrium states emerges in the energetic landscape [9] . When this happens, replicas of the system, such as identical copies under the same experimental conditions, may furnish different values of observable quantities, because they settle in ergodically separated states after a long dynamics. This phenomenon is inherently different from chaos, and relies on non-trivial equilibrium properties of disordered systems. RLs are realized in disordered media with gain; the feedback for stimulated emission of light is given by the scattering and no external cavity is needed [10] . Different RLs show multiple sub-nanometer spectral peaks above a pump threshold [11] . The wide variety of the spectral features reported and the still debated emission properties are due to the fact that RLs are open systems where light can propagate in any direction in a disordered manner instead of oscillating between well specific boundaries as in standard lasers [12] . The scattering strength and pumping conditions [13] , [14] , [15] , [16] , [17] affect the emission: a large number of modes may result in a continuous broadband, or exhibit distinguishable resonances. Various authors have reported evidences of shot-to-shot fluctuations in RLs. In the study by Fallert et al. [18] they are ascribed to the coexistence of localized and extended modes without analyzing the statistical distribution of their shot-to-shot correlations. In the study by van der Molen et al. [19] they are due to the intrinsic matter fluctuations in fluids that are not present in samples with static disorder as in the case here considered. In the study by Lepri et al. [20] the analysis of the different diffusion regimes is reported and it is not linked to a phase transition from spontaneous emission to RL, because the exponent of the diffusion law does not help to discriminate lasing from fluorescence. In the study by Mujumdar et al. [21] mode-competition and seemingly chaotic behaviour have been considered and intended as a generic sensitivity to initial conditions, no analysis of the distribution of the shot-to-shot correlations is provided. In the study by Skipetrov et al. [22] fluctuations due to a transparent Kerr medium are theoretically considered, and even if they are not strictly related to the case with gain and loss of RLs, they look to have connections with the spin-glass approach in the study by Leuzzi et al. [6] , [7] , [8] The latter approach has been developed in a series of papers, and is based on the mode-coupling laser theory as, for example, in the study by Leonetti et al. [23] , which reports on the time dynamics of frequency locking mechanism and without addressing the statistical properties of the laser emission. Our understanding is that the RL spectral fluctuations are a manifestation of the existence of many degenerate lasing states, each one corresponding to a given ensemble of activated modes with their own wavelengths, phases and intensities. This theory is a statistical mechanical formulation obtained starting from the decomposition in normal modes of the electromagnetic field of light, in the presence of nonlinearity, and leading to a quenched disordered spin-glass-like Hamiltonian. The theoretical approach considers the combined effect of localized and radiating modes as occurring in any open cavity, and allows to describe open systems with arbitrary degree of openness [8] . A complex landscape typical of glassy systems is expected to occur beyond some threshold critical value of the external parameter driving the transition. The measurements reported in this manuscript confirm this theory: in a system that might be properly represented by a spin-glass theory [6] , [7] , [8] we measure the spin-glass order parameter distribution function, such as P ( q ) and we find a behaviour akin to the one theoretically representing the spin-glass phase (at high pumping) and the paramagnetic/fluorescence phase (at low pumping), as well as the transition between them. Spin-glass theory of RLs In the following, we report on the shot-to-shot emission fluctuations from planar RLs made of a fluorescent π-conjugated oligomer in amorphous solid phase and we analyze the experimental results by means of the replica theory. At variance with standard chaotic ordered lasers [24] , [25] , in which, for specific and tailored conditions, few modes provide exponentially diverging temporal trajectories, RLs are thermodynamic systems, with thousands of modes and degrees of freedom, which exhibit a huge number of (meta-)stable states. A standard chaotic laser will always display the same spectral behaviours in the same conditions; at large variance with what we observe in RLs. In the spin-glass approach the RL modes are treated as continuous complex spin variables with a global (power) constraint and whose coupling is governed by the interplay between disorder and nonlinearity. We remark that in this theoretical analysis, the Hamiltonian description is an effective one, representing the stationary regimes under pumping. The role of inverse temperature in equilibrium thermodynamics is played by the energy pumped into the system. The Hamiltonian description is derived in such a way to encode, in a distinct, effective temperature space, pumping and dissipation of the laser. Hence, the theoretical approach also includes the fact that RLs are open dissipative systems with an external pumping mechanism and radiation losses [8] . In our experiments the disorder is fixed and the nonlinearity increases with the pumping energy, which acts as the inverse of temperature in statistical mechanics [26] , [27] : at low energy (high temperature) there is no gain competition [28] , [29] between the modes and they oscillate independently in a continuous wave paramagnetic regime, while at high energy (low temperature) the coexistence of mode coupling through the gain competition and frustration due to disorder gives rise to a glassy regime. In this regime, a large number of electromagnetic modes is activated and in interaction. The set of the activated mode configurations is found to change from pulse-to-pulse. We will refer to each set of configurations as a state. This is justified by the fact that during a single pulse of the pump beam, very many stimulated emission processes take place at each mode frequency, that is, each mode performs a long dynamics, compatible with thermalization. The observation of numerous different states can be understood as the evidence of a thermodynamic phase corresponding to many valleys separated by barriers in the corrugated free energy landscape. The same sample under identical experimental conditions furnishes different laser emissions. Each different instance of laser emission is, thus, a physical realization of a replica, in the meaning introduced in replica theory [1] . RL emission The investigated system is a functionalized thiophene-based oligomer commonly named thienyl-S,S-dioxide quinquethiophene (T5OCx; see Methods for details) in amorphous solid state, as shown in the confocal microscopy image reported in Fig. 1a . RL in T5COx spin-coated in thin films [30] and lithographed in micro-structures [31] has been previously observed. The strong density of the T5OCx supra-molecular laminar packing in the solid samples allows to study shot-to-shot emission fluctuations not reported so far. A sketch of the pumping and collecting geometry is given in the inset of Fig. 1b . Experimental details are reported in Methods. 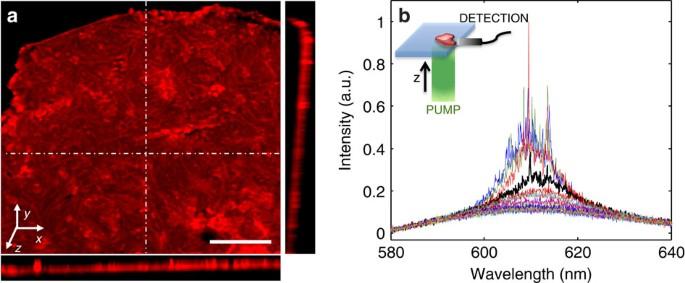Figure 1: Sample image and emission spectra showing random lasing. (a) Three-dimensional-reconstruction of confocal microscopyz-stack images of the supra-molecular laminar packing in aT5OCx solid sample. The right and the bottom panels report theyz- and thexz- sections, respectively. Scale bar, 20 μm. (b) High resolution single shot spectra taken in the same conditions, 10 mJ pump energy. Inset: sketch of the experiment. Figure 1: Sample image and emission spectra showing random lasing. ( a ) Three-dimensional-reconstruction of confocal microscopy z -stack images of the supra-molecular laminar packing in aT5OCx solid sample. The right and the bottom panels report the yz - and the xz - sections, respectively. Scale bar, 20 μm. ( b ) High resolution single shot spectra taken in the same conditions, 10 mJ pump energy. Inset: sketch of the experiment. Full size image We illustrate in Fig. 1b , single shot high resolution (0.07 nm) emission spectra, taken at identical experimental conditions. Input energy is 10 mJ. The presence of RL modes with configuration variable from pulse-to-pulse is evident: each time the system is pumped the numerous passive modes randomly compete for the available gain, giving rise to several different compositions of the activated spectral peaks [21] . Such behaviour is also evidenced by the direct visualization of the sample during pumping, as reported in Fig. 2 , where four different fluorescence images taken at four single shots exhibit different emission patterns and corresponding spectral features. It is clear that from shot-to-shot the intensity and the profile of the bright spots, where the RL modes are concentrated, change. Each bright spot contains many interacting modes as evidenced by the spectra with many peaks and by the size of the spots. Many extended modes are concentrated in different extended spots and from shot-to-shot the size and the brightness of these spots change showing that the spatial structure of the modes changes. 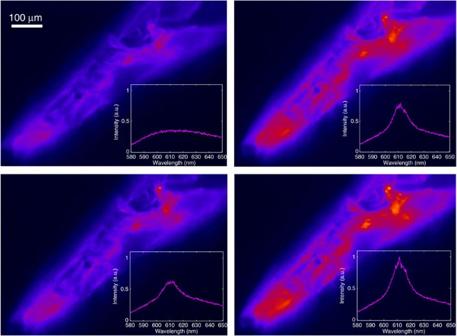Figure 2: Snapshots of RL emissions. Optical images and corresponding emission spectra (insets) during the pumping of the sample in the same experimental conditions. The input energy is 10 mJ. Figure 2: Snapshots of RL emissions. Optical images and corresponding emission spectra (insets) during the pumping of the sample in the same experimental conditions. The input energy is 10 mJ. Full size image In Fig. 3a,b we show emissions of subsequent 100 shots with lower spectral resolution (0.3 nm), at two different pump energies. There is no time periodicity in the spectral fluctuations: their sequence is random. At low energy, the noisy variations of the spontaneous emission are negligible if compared with the pronounced fluctuations observed at high energy. 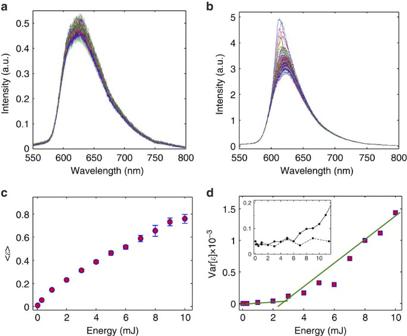Figure 3: Fluctuations in the random laser emission. (a,b) Emission spectra at low energy 1 mJ (a) and high energy 10 mJ (b). (c) Mean emission intensity <ε> versus pump energy, error bars are s.d. (d) Variance ofεversus pump energy. Inset: peak s.d. divided by mean peak intensity from the sample (solid line) and the pump laser (dashed line) emission spectra. Figure 3: Fluctuations in the random laser emission. ( a , b ) Emission spectra at low energy 1 mJ ( a ) and high energy 10 mJ ( b ). ( c ) Mean emission intensity < ε > versus pump energy, error bars are s.d. ( d ) Variance of ε versus pump energy. Inset: peak s.d. divided by mean peak intensity from the sample (solid line) and the pump laser (dashed line) emission spectra. Full size image Analysis of the spectral emissions The cavity coupled modes in the Hamiltonian describing RLs [6] are variables not easily accessible in the experiments. We can otherwise measure spectra and have access to the intensities , where a j is the amplitude of the longitudinal mode j (refs 6 , 7 ) at wavelength λ j . In our analysis each spectrum represents a different state of the same thermodynamic phase. The average is taken over all modes having similar wavelength, binned together in data acquisition with index k , due to the finite spectral resolution Δ λ =0.3 nm. We define the average spectral intensity as α being the replica index and N the number of acquired spectral points. The variation of this parameter from shot-to-shot quantifies the observed fluctuations. Mean and variance of ε α over N s replicas for each pumping are Figure 3c shows the continuous growth for increasing input energy of the mean intensity, equation (2). It is very important to explain the stimulated emission we are observing. In our samples we see the coexistence of RL and amplified spontaneous emission (ASE) [30] , [32] . The latter is evident from the absence of threshold in the spectral peak intensities in Fig. 3c and RL is evident from the fine peaks superimposed to the ASE band in Fig. 1b . This specific system, made of thick amorphous solid dye, displays a threshold in terms of the spectral fluctuations, quantified by Var[ ε ], calculated as equation (3) and shown in Fig. 3d . Such behaviour has not been reported in previous works on similar dyes [30] , [32] . It is well-known that ASE does not exhibit a threshold, at variance with RL. However, in our case, the RL threshold is masked by ASE when coming at the spectral peak. On the contrary, the threshold of the fluctuations in Fig. 3d reveals the onset of the RL action, that for this sample is estimated around 3 mJ. All experiments are performed in the same environmental conditions, that is the temperature, the position and the state of the sample and the performances of the optical components are controlled to be stable by growing pump energy. To check the stability of the input laser, we estimate the energy fluctuations as the percentage variation given by the ratio between the s.d. and the mean value of the emission peak intensity with and without sample, for increasing energy. The plots are reported in the inset of Fig. 3d , where the laser energy variations are ~4% at any energy, while the same quantity from the sample increases at high energy. We stress that an error of 4% on the x -axis of Fig. 3d is inside the symbols and negligible compared with the energy values, thus it cannot cause the evident increase of the observed variance. To analyze the system behaviour in the framework of statistical mechanics of disordered systems and characterize the high pumping RL regime, we introduce another order parameter to identify the phase transition: the overlap between intensity fluctuations in different experimental replicas. The experimentally accessible variable, coarse graining the behaviour of single modes, is the intensity fluctuation at a given frequency: with Ī ( k ) the average over replicas of each mode intensity The overlap between pulse-to-pulse intensity fluctuations is defined as From the measured spectra we calculate the set of all N s ( N s −1)/2 values q of q αβ for each different input energy, determining their distribution P ( q ). We retain P ( q ) as a measure of the theoretical distribution of the overlap between mode amplitudes [6] , [7] , which is a leading quantity for the description of glassy phases [1] . So far no experimental measurements of P ( q ) have been reported. Six examples are reported in Fig. 4a–f for increasing pump energy. At low energy ( Fig. 4a ), all overlaps are centred around the zero value, meaning that the electromagnetic modes are independent and do not interact in the paramagnetic regime. By increasing energy, modes are coupled by the nonlinearity and this corresponds to a non-trivial overlap distribution ( Fig. 4b–f ). In the high energy glassy phase, with all modes highly interacting and frustrated by the disorder, q assumes all possible values in the range [−1,1]. Such behaviour of the P ( q ) evidences the fact that the correlation between intensity fluctuations in any two replicas depends on the replicas selected. The variety of possible correlations extends to the whole range of values. This is a manifestation of the breaking of the replica symmetry. In Fig. 4g , we show q max corresponding to the position of the maximum of P (| q |) versus pumping: it changes drastically signalling a phase transition between 2 and 3 mJ, compatible with the threshold determined by Var[ ε ] in Fig. 3d . We point up that in the high pump regime P ( q )>0 for any value of q . 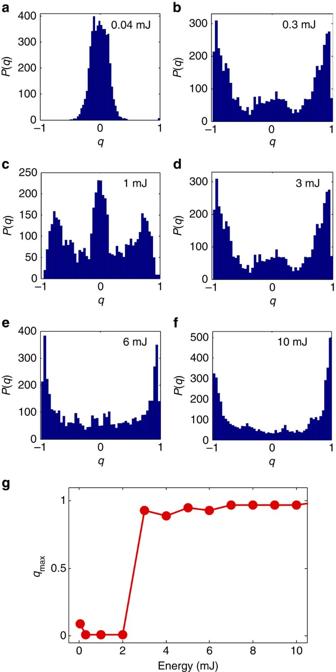Figure 4: Distribution function of the overlap showing replica symmetry breaking by increasing pump energy. (a–f) Distribution of the overlapqat different pump energy. (g)qmaxcorresponding to the position of the maximum ofP(|q|) versus pumping. Figure 4: Distribution function of the overlap showing replica symmetry breaking by increasing pump energy. ( a – f ) Distribution of the overlap q at different pump energy. ( g ) q max corresponding to the position of the maximum of P (| q |) versus pumping. Full size image To stress the peculiarity of such a signature of RSB and the relevance of the analysis method proposed in probing the onset of a prominent glassy nature of RL regimes in different compounds, we compare the different behaviour of P ( q )’s generated by an identical analysis for the emission spectra of a standard ordered laser, the same used as pump laser in the experiments, as reported in Fig. 5a , and of a differently structured RL, a liquid dispersion of titanium dioxide in 3 mM rhodamine B-ethylene glycol solution, shown in Fig. 5c,e,g . In Fig. 5b , the standard laser (obviously well above threshold) does not show any symmetry breaking, even though small fluctuations are present, as expected in an ordered system. In Fig. 5d,f,h , the P ( q )’s for the liquid RL are displayed by increasing pump energy across its estimated threshold of 0.25 mJ and no evident signs of RSB above the lasing threshold can be appreciated up to 0.85 mJ. This result points out that indications about the occurrence of RSB depend on the characteristics of the system and are, therefore, a way to classify the nature of different RLs. 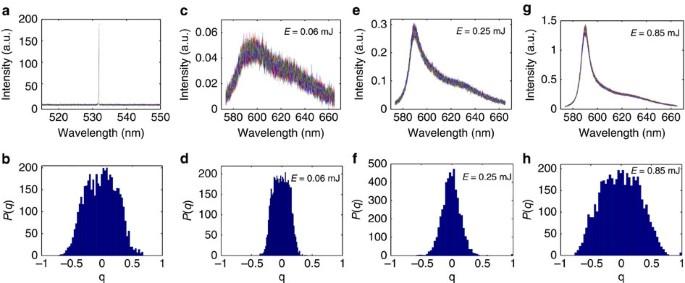Figure 5: Distribution function of the overlap in standard and random laser without replica symmetry breaking. (a,b) Emission spectra (a) andP(q) (b) of a Q-switched pulsed Nd-Yag standard ordered laser. The analysis is done on 100 shots. (c–h) Emission spectra (c,e,g) and correspondentP(q) (d,f,h) of a liquid dispersion of titanium dioxide in rhodamine B-ethylene glycol solution at three different pump energy through the threshold. Figure 5: Distribution function of the overlap in standard and random laser without replica symmetry breaking. ( a , b ) Emission spectra ( a ) and P ( q ) ( b ) of a Q-switched pulsed Nd-Yag standard ordered laser. The analysis is done on 100 shots. ( c – h ) Emission spectra ( c , e , g ) and correspondent P ( q ) ( d , f , h ) of a liquid dispersion of titanium dioxide in rhodamine B-ethylene glycol solution at three different pump energy through the threshold. Full size image We experimentally show that the RL intensity fluctuations in a solid disordered system grow drastically as the pump energy increases beyond a threshold, exhibiting a transition from negligible to large oscillations. A possible order parameter is quantified by the variance of the fluctuations. A more refined one is the distribution of all mutual overlaps between intensity fluctuations in different physical replicas. Besides evidencing the threshold of phase transition, it describes the organization of states and their non-trivial correlation, nonsymmetric in replicas exchange. Above the threshold pump energy, the overlap between two replicas does depend on the specific couple chosen and the variation from couple to couple turns out to be more complicated than the ordinary statistical fluctuations. That is, replicas are not all equivalent to each other in the analyzed RL and we, thus, observe an instance of RSB through the RL transition. The parameter q measures the overlap of the shot-to-shot fluctuations at each wavelength around the average spectrum at a given pumping. Thus q ~1 when two shots have very similar intensity fluctuations at each wavelength. In principle, it does not matter how large the fluctuations are to have a large q , but only how much they are correlated. The fact that large overlap values become probable in the lasing regime above threshold is not a trivial feature. Similarly, one has q ~−1 when two shots display spectral fluctuations similar in magnitude (no matter how large) but opposite in sign, that is the shot-to-shot fluctuations around the average spectrum are very anti-correlated. When q ~0, the intensity fluctuations in two shots are basically uncorrelated. This can imply the ASE background, but can also correspond to the presence of a subset of shots with uncorrelated large fluctuations. Above threshold, the latter situation occurs, as can be observed looking at the single spectra. By the definition of overlap in equation (6), in all cases | q |~[0, 1], the fluctuations of a single spectrum can be large or small. The important observation is that increasing the pumping, the correlations between shot-to-shot fluctuations become non-trivial right when the fluctuation magnitude starts increasing significantly (such as above threshold), see Fig. 3d . In the present work not only a first experimental proof of RSB is presented, but a new method is provided that allows to characterize the nature of the randomness above the lasing threshold applicable to the whole profusion of RLs. By directly probing the measure of spectral intensity fluctuations, the possible existence and the organization of many equivalent competing lasing states yielding a glassy light behaviour can be verified, allowing for an alternative, supplementary RL classification in terms of glassiness. As a last remark, we recall that in the effective statistical mechanical Hamiltonian for RLs the variables are, actually, the modes, such as complex amplitudes [6] , [7] , [8] , not easily accessible in the experiments, whereas we are considering their squared modulus given by the emitted intensity, thus losing information about the actual state structure. Looking at the present results we stress, however, that such coarse graining appears to be refined enough to investigate the peculiar properties of glassy-like regimes of RLs. Sample preparation and characterization The investigated disordered system is a functionalized T5OCx, whose preparation modalities and molecular structure are reported elsewhere [31] , in amorphous solid state obtained by the crystallization of the dye powder after a thermal shock above the transition temperature ( T g ). Successively, the packing states have been frozen by cooling across the T g . The thermal process confers to the π-conjugated oligomer a crystal-like molecular ordering over large area with the appearance of laminar domains that grow anisotropically in time up to their final random packing leading, at the end of the process, to a macroscopic disordered system as shown in Fig. 1a . Sample characterization is performed by a z -stack sequential acquisition of confocal microscope (Olympus, FV1000). The optical sections are collected in transverse xz - and yz - planes. The x – y surface area of the investigated samples is in the range (10 5 –10 6 ) μm 2 and the average thickness along z is (7±2) μm. Measurements The samples are pumped by a frequency doubled Q-switched Nd:YAG pulsed laser emitting at λ =532 nm, with 10 Hz repetition rate, 6 ns pulse duration and with 12 mm beam diameter, the emitted radiation is collected from the sample edge into an optic fibre connected to a spectrograph equipped with electrically cooled CCD array detector, with grating densities of 600 and 1,800 mm −1 , for low (0.07 nm) and high (0.3 nm) resolution spectra, respectively. The spectral acquisition is triggered by the pump laser flash lamp at 10 Hz repetition rate. The samples are put on glass slides and pumped perpendicularly along the z direction and all reported spectra are taken from single pumping shots. In Fig. 2 the transmitted fluorescence is imaged on a CCD camera (along z axis) by a microscope objective with numerical aperture 0.75. How to cite this article: Ghofraniha, N. et al. Experimental evidence of replica symmetry breaking in random lasers. Nat. Commun. 6:6058 doi: 10.1038/ncomms7058 (2015).